A bi-functional device for self-powered electrochromic window and self-rechargeable transparent battery applications Electrochromic smart windows are regarded as a good choice for green buildings. However, conventional devices need external biases to operate, which causes additional energy consumption. Here we report a self-powered electrochromic window, which can be used as a self-rechargeable battery. We use aluminium to reduce Prussian blue (PB, blue in colour) to Prussian white (PW, colourless) in potassium chloride electrolyte, realizing a device capable of self-bleaching. Interestingly, the device can be self-recovered (gaining blue appearance again) by simply disconnecting the aluminium and PB electrodes, which is due to the spontaneous oxidation of PW to PB by the dissolved oxygen in aqueous solution. The self-operated bleaching and colouration suggest another important function of the device: a self-rechargeable transparent battery. Thus the PB/aluminium device we report here is bifunctional, that is, it is a self-powered electrochromic window as well as a self-rechargeable transparent battery. Energy saving and CO 2 emission reduction are becoming more and more urgent because of pressing issues such as global warming, climate change and resultant environmental concerns. In line with these worldwide efforts, use of smart windows will significantly decrease the cost of air conditioning and sun shading, and simultaneously improve the indoor comfort with added decoration effect [1] . Though photochromic [2] and thermochromic [3] technologies can also be used for smart windows, electrochromic (EC) smart windows [4] , [5] , [6] , [7] , [8] which can reversibly change their colours under external biases, own advantages with much better controllability, energy saving and durability. However, conventional EC devices need external biases to operate, resulting in additional energy consumption. Meanwhile, significant progress has been made on photovoltaic-powered EC (PV-EC) [9] and photoelectrochromic (PEC) devices [10] . By using these technologies, external wiring and power sources are not necessary in theory. However, the switching of PV-EC and PEC devices is weather dependent, often resulting in an unsatisfied controllability. As a result, PV-EC and PEC devices are still connected with external power sources in practice. Moreover, use of photovoltaics increases the cost and incurs more reliability issues. Consequently, an easily controllable and low-cost self-powered EC device, which can be used whenever and wherever, is much desired; however, this still remains challenging until now. On the other hand, lithium ion battery, one of the most popular energy storage devices, is attracting considerable interest in cell phones, laptop computers, electric vehicles, lighting, military and aerospace applications due to its high energy density, long lifetime and small size [11] , [12] , [13] , [14] . In general, charging of batteries consumes electricity. Thus far, there is a lack of battery electrodes that can be self-recharged utilizing some spontaneous chemical reactions in ambient conditions. EC materials, capable of storing/releasing ions and electrons in switching, have been previously studied to show battery characteristics [15] , [16] . As one of known EC materials, iron(II,III) hexacyanoferrate(II,III), commonly known as Prussian blue (PB), is a coordination compound and has long been used as a blue pigment [17] , [18] , [19] , [20] . The application of PB as an EC material was pioneered by Neff and coworkers [21] , [22] and Itaya et al. [23] , [24] , [25] PB can be reduced to colourless ‘Everitt’s Salt’ (Prussian white (PW)), oxidized to Berlin green and ‘Prussian yellow’ by electrochemical reactions [21] , [26] . Neff [27] also studied a PB battery in which both the anode and cathode are PB films electrochemically deposited on porous graphite, and an improved battery using PB and Nafion composite was also reported by Honda et al. [28] However, the Neff cell has a low theoretical output voltage of 0.68 V, and the voltage of the charged battery continually drops in air due to the oxidation of PW to PB. The low voltage drawback cannot be overcome for Neff cells (using EC films for both anode and cathode) even employing PB analogues, such as zinc hexacyanoferrate/PB and copper hexacyanoferrate/PB [29] . Moreover, these cells cannot be used as EC smart windows because the two EC films employed cannot simultaneously change their colours due to opposite biases applied. Recently, Cui and co-workers [30] reported a lithium battery using copper hexacyanoferrate mixed with carbon as the electrode material. A similar electrode material of iron hexacyanochromate has also been used as an anode material for rechargeable batteries [30] . In brief, all the above-mentioned batteries [27] , [28] , [29] , [30] , [31] do not utilize the EC function of these EC materials, and their output voltage is relatively low. Like conventional batteries, they are not self-rechargeable and the charging relies on an external power source. The colouration from PW to PB corresponds to the oxidation of Fe(II) (a low oxidation state of Fe in PW) to Fe(III) (a higher oxidation state of Fe in PB), which can spontaneously take place in an aqueous solution containing dissolved oxygen [19] , [32] . It is thus possible to realize a self-rechargeable battery by reducing PB to PW during discharge, if one can find a suitable material, which can easily lose electrons and has a large electrode potential difference with PB for a high output voltage. Considering the strong reducing capability of Al, Al and PB should be a good combination for a high-voltage battery, supplying the driving potential for bleaching PB itself. In this work, we demonstrate a bi-functional PB/Al device for self-rechargeable battery and self-powered EC device applications. As a self-powered EC device The device consists of a PB film electrochemically deposited on a piece of indium tin oxide (ITO) coated glass (the PB electrode) and a strip of Al sheet attached on another piece of ITO glass (the Al electrode) using 3 mol l −1 KCl aqueous electrolyte. Considering the application of the device as an EC smart window, the strip of Al sheet is attached onto only one side of the ITO glass, which leaves most area of the as-prepared device transparent. The original blue colour ( Fig. 1a ) of the device is from the PB film. Without applying any external bias, the blue device can be quickly bleached to colourless ( Fig. 1b ) by connecting the PB and Al electrodes (a video for the self-bleaching of the device is available in Supplementary Video 1 ). The corresponding transmittance change is shown in Fig. 1c . The maximum optical modulation of the device is 52.2% at 670 nm, which is actually high enough considering that light has to go through two sheets of ITO glass and electrolyte. A similar phenomenon was observed when replacing Al with Fe ( Supplementary Fig. 1 ), clearly implying that the colour bleaching of the device is related to the reduction of PB by strongly reducing metals. 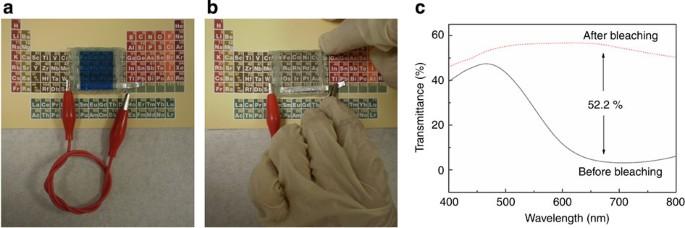Figure 1: Characterization of the self-powered PB/Al EC device. (a) Optical photo of the as-prepared EC device. (b) The bleached state by connecting the PB and Al electrodes, and (c) the corresponding transmittance change of the EC device. Figure 1: Characterization of the self-powered PB/Al EC device. ( a ) Optical photo of the as-prepared EC device. ( b ) The bleached state by connecting the PB and Al electrodes, and ( c ) the corresponding transmittance change of the EC device. Full size image The bleached device can spontaneously recover its blue colour by disconnecting the PB and Al electrodes, as shown in Fig. 2a,b (the bleaching and recovery of PB film in a beaker is shown in Supplementary Fig. 2 ). This is quite interesting because it means that the as-prepared PB/Al cell can be used as a self-powered EC device; the bleaching is realized by connecting the PB and Al electrodes and subsequent colouration is achieved by the spontaneous recovery. The transmittance change ( Fig. 2c ) of the bleaching/colouration (recovery) switching of the self-powered EC device was measured in situ using an ultraviolet–visible spectrophotometer by connecting the working PB electrode and Al electrode for 10 s and then disconnecting for 590 s for the recovery of the device. The transmittance is increased by 43.9% in the first 10 s (connecting PB and Al electrodes) and decreased by 21.3% in the next 590 s (disconnecting PB and Al electrodes), showing a characteristic of fast bleaching and slow colouration (recovery). For 90 and 70% transmittance changes (within the total 43.9% transmittance change obtained in the first 10 s), the corresponding bleaching times are only 3.3 and 2.3 s, respectively. 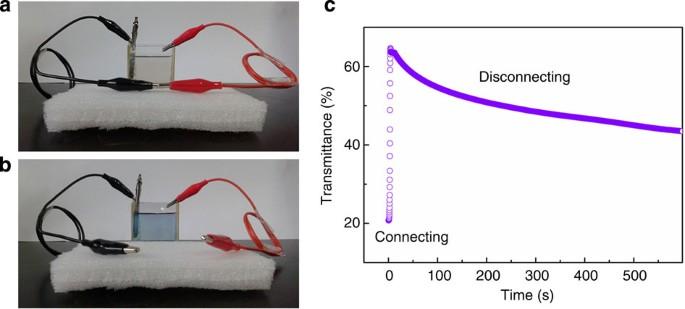Figure 2: Characterization of the colour restoration process of the PB/Al EC device. (a) Optical photo of the bleached EC device, and (b) the EC device recovered for 1 h. (c)In situtransmittance measurement of the EC device connected for the first 10 s and then disconnected for next 590 s. Figure 2: Characterization of the colour restoration process of the PB/Al EC device. ( a ) Optical photo of the bleached EC device, and ( b ) the EC device recovered for 1 h. ( c ) In situ transmittance measurement of the EC device connected for the first 10 s and then disconnected for next 590 s. Full size image The transmittance spectra for the progressive recovery of the bleached device are shown in Fig. 3a . At 670 nm, the transmittance of the device is decreased by 15.7, 22.4, 29.2, 38.5 and 45.8% after a recovery time of 5, 15 min, and 1, 2, and 4 h, respectively, showing a gradually decreasing colouration rate (or recovery rate). The transmittance decrease within the first 5 min is more than that of the next 55 min. Within the first 2 h, the transmittance change is 38.5%. However it is only 7.3% for the next 2 h. Besides the spontaneous recovery, the as-prepared PB/Al cell can also be coloured by an external bias, which will greatly accelerate the colouration rate. By alternately connecting the PB and Al electrodes for 10 s and applying an external bias of 2 V for 10 s, the PB/Al cell is reversibly switched between high and low transmittances, as shown in Fig. 3b . The recoverable high and low transmittance implies good reversibility of the bleaching/colouration switching processes. The calculated bleaching and colouration time is 4.1 and 4.6 s, respectively. 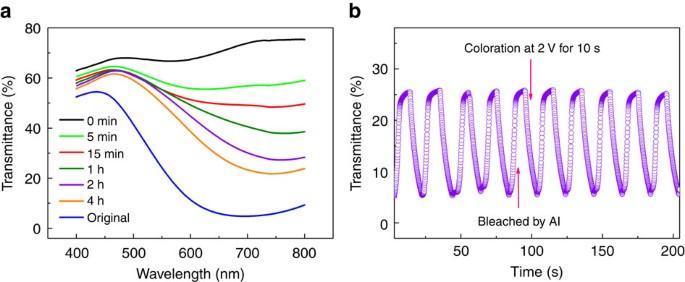Figure 3: Spontaneous colour restoration and reversible bleaching/colouration switching. (a) Transmittance spectra of the original self-powered PB/Al EC device (original curve) and the bleached device at various recovery times from 0, 5 min to 4 h. (b) Reversible bleaching/colouration switching driven by alternately connecting the Al and PB electrodes for 10 s and supplying an external bias of 2 V for 10 s. Figure 3: Spontaneous colour restoration and reversible bleaching/colouration switching. ( a ) Transmittance spectra of the original self-powered PB/Al EC device (original curve) and the bleached device at various recovery times from 0, 5 min to 4 h. ( b ) Reversible bleaching/colouration switching driven by alternately connecting the Al and PB electrodes for 10 s and supplying an external bias of 2 V for 10 s. Full size image As a self-rechargeable battery Another interesting function of the as-prepared self-recoverable PB/Al cell is its potential use as a self-rechargeable battery. The measured open circuit potential of the PB/Al battery with 3 mol l −1 KCl electrolyte is 1.26 V, which is significantly higher than that of previously reported EC materials-based batteries [27] , [28] , [29] . To light up a red light-emitting diode (LED), we connected two PB/Al cells in series, which can supply a voltage of 2.52 V. The LED is brightest when powered by the freshly prepared cells ( Fig. 4a,b ) (the corresponding videos are available in Supplementary Videos 2 and 3 ). 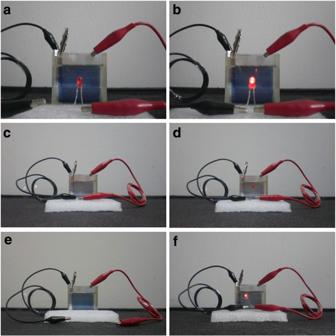Figure 4: Photos of the as-prepared two PB/Al devices connected in series acting as self-rechargeable batteries. (a) In coloured state with two electrodes disconnected, and (b) the connected circuit powering a LED. (c) In bleached state with connected PB electrode and Al electrode, and (d) connected circuit showing no light from the LED. (e) After recovering for 1 h with circuit disconnected, and (f) connected circuit powering the LED. Figure 4: Photos of the as-prepared two PB/Al devices connected in series acting as self-rechargeable batteries. ( a ) In coloured state with two electrodes disconnected, and ( b ) the connected circuit powering a LED. ( c ) In bleached state with connected PB electrode and Al electrode, and ( d ) connected circuit showing no light from the LED. ( e ) After recovering for 1 h with circuit disconnected, and ( f ) connected circuit powering the LED. Full size image After being bleached to colourless ( Fig. 4c ), the LED cannot be lighted up ( Fig. 4d ), implying the discharged state in the bleached device. However, after disconnecting the PB and Al electrodes for 1 h, the PB/Al cells are recovered to bluish ( Fig. 4e ) and able to light up the LED again ( Fig. 4f ), indicating that the battery was partially recharged. The recovery from colourless to blue colour of the PB/Al cell corresponds to the charging process of the battery; a deeper colour means a higher charging extent. In this sense, the amount of stored electricity of the self-rechargeable PB/Al battery can be clearly indicated by its colour. The discharge process (as a battery) of the PB/Al cell corresponds to its bleaching process (as an EC device). The amount of charge (that is, battery capacity) involved during the discharge process and the subsequent charge (colour restoration in the EC device) process can be accurately measured by an electrochemical workstation. 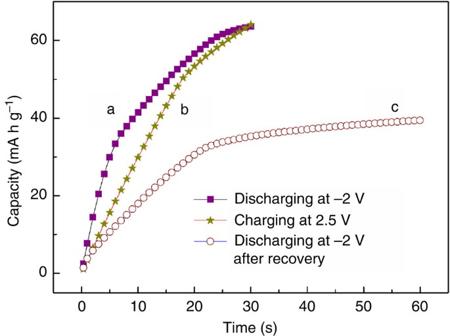Figure 5: Specific capacities of the original and recovered PB/Al cells. (a) Discharging capacity curve at −2 V, and (b) charging capacity curve at 2.5 V for the original PB/Al cell and (c) discharging capacity curve at −2 V for the recovered PB/Al cell with a 24 h recovery in air. Figure 5 shows the specific accumulative discharge and charge capacity of the original and recovered PB/Al cells. The discharge capacity at −2 V for 30 s is 63.6 mA h g −1 ( Fig. 5a ) and the charge capacity at 2.5 V for 30 s ( Fig. 5b ) is 64.1 mA h g −1 , which are comparable to the capacity of recently reported copper hexacyanoferrate battery [29] . The discharge and charge capacities are very close, implying a good reversibility in the charging/discharging of the as-prepared PB/Al battery. After spontaneous recovery for 24 h, the recovered PB/Al battery is able to deliver a discharge capacity of 39.4 mA h g −1 ( Fig. 5c ), that is 61.9% of the total dischargeable amount of the original PB/Al cell. Though the specific capacity is relatively low compared with those of lithium batteries [11] , [12] , [13] , [14] , the as-prepared PB/Al battery is potentially capable of providing a reasonably large total capacity in a limited volume and a high voltage with the thin-layered structure. If an external bias is applied to charge the bleached device instead of self-charging in air, both of the charge and re-discharge capacities can be increased by ~27.8% ( Supplementary Fig. 3 ). Figure 5: Specific capacities of the original and recovered PB/Al cells. (a) Discharging capacity curve at −2 V, and (b) charging capacity curve at 2.5 V for the original PB/Al cell and (c) discharging capacity curve at −2 V for the recovered PB/Al cell with a 24 h recovery in air. Full size image Further battery characterizations We further characterize the battery characteristics of the PB/Al cell. The cyclic voltammetric response of the PB film electrode is first investigated using a three-electrode system ( Supplementary Fig. 4 ), in which the PB film on ITO was used as the working electrode and the Al foil and standard calomel electrode (SCE) were used as the counter electrode and the reference electrode, respectively. The measured open circuit potential of the half cell is 0.4 V versus SCE. Consistent with a previous report, the cyclic voltammetric behaviour is accompanied by two redox couples in accordance with the following reactions [33] : Reaction (1) with a potential of 0.18 V versus SCE (the first pair of peaks) is referred to the reduction of PB to PW via one-electron transfer to the low-spin iron atom. Reaction (2) at 0.96 V versus SCE is referred to the oxidation of PB to so-called ‘Berlin green’ (BG) via one-electron transfer oxidizing high-spin iron in PB lattice. As for the two-electrode PB/Al cells (that is, Al foil served as both the counter electrode and the reference electrode), the cell reaction is only related with the bleaching and recovery of PB. Considering the potential difference of Al versus SCE (−0.86 V), the bleaching process might occur around 1.0 V (that is, 0.18+0.86 V). Meanwhile, the potential corresponding to the oxidation of PW to PB might shift to even higher position to overcome the overpotential. Herein, the electrochemical measurements using the two-electrode configuration are performed in a wider voltage range between 0.8 and 2.1 V to focus on the redox reactions between PB and PW. The cyclic voltammetric response of the PB/Al cell is shown in Fig. 6a . One pair of peaks (cathodic, anodic) observed at the potentials (V) of (1.0, 1.9) can be attributed to the reduction of PB to PW (cathodic scan) and oxidation of PW to PB (anodic scan). In agreement with the CV result, one charge plateau (~1.9 V) and one discharge plateau (~1.1 V) can be observed in the charge/discharge curves, which can be assigned to the Fe(III)/Fe(II) redox couple in PB and PW ( Fig. 6b ). The initial discharge and charge capacities are 72.2 mA h g −1 and 72.1 mA h g −1 , respectively. 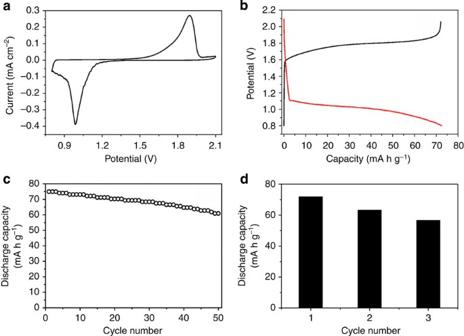Figure 6: Electrochemical properties of PB/Al cells. (a) The cyclic voltammogram at a scan rate of 5 mV s−1using a two-electrode configuration. (b) Galvanostatic discharge and charge curves of the PB/Al cell at a current density of 2000, mA g−1. (c) Cycling performance of the PB/Al cell. (d) Repeated self-rechargeability test of the PB/Al cell with a 12 h recovery in deionized water bubbled with O2gas (~100 ml min−1). Figure 6c shows the discharge–charge cycling performance evaluated between 0.8 and 2.1 V using the two-electrode configuration. When cycled at a current density of 2000, mA g −1 , a capacity of 75 mA h g −1 is obtained in the first cycle, and 81% of this capacity (61 mA h g −1 ) can be retained after 50 cycles. Moreover, the PB films can deliver higher capacities at a lower current density of 400 mA g −1 ( Supplementary Fig. 5 ). The spontaneous self-recharging process of the PB/Al cell was investigated with a 12-h recovery in deionized water bubbled with O 2 gas. After cycling for three times, the recovered PB/Al battery can still deliver a discharge capacity of 56.6 mA h g −1 ( Fig. 6d ), with a total capacity loss of 20% compared with the first discharge process (71.9 mA h g −1 ). Furthermore, the internal resistance of the cell was investigated through the electrochemical impedance spectroscopy measurements ( Supplementary Fig. 6 ). The cell behaves like a resistance at high frequencies. Whereas, the imaginary part of the impedance sharply increases and the plot appears to be a vertical line characteristic of capacitive behaviour at low frequencies [34] . A possible explanation of the high resistance shown by the cell with the decreasing frequency might be related to the high impedance of the electrolyte [30] , [35] . Figure 6: Electrochemical properties of PB/Al cells. ( a ) The cyclic voltammogram at a scan rate of 5 mV s −1 using a two-electrode configuration. ( b ) Galvanostatic discharge and charge curves of the PB/Al cell at a current density of 2000, mA g −1 . ( c ) Cycling performance of the PB/Al cell. ( d ) Repeated self-rechargeability test of the PB/Al cell with a 12 h recovery in deionized water bubbled with O 2 gas (~100 ml min −1 ). Full size image The functioning mechanisms of self-powered EC device and self-charging battery are schematically illustrated in Fig. 7 . Al is an active metal, which easily releases electrons to form Al 3+ ions, whereas PB can act as an oxidant to acquire electrons by the reduction of Fe(III) to Fe(II), accompanied by the insertion of charge-balancing K + ions from electrolyte when PB and Al electrodes are connected ( Fig. 7a ). The mechanism for the bleaching (as a self-powered EC device, see Fig. 7a,b ) or discharging (as a self-rechargeable battery, see Fig. 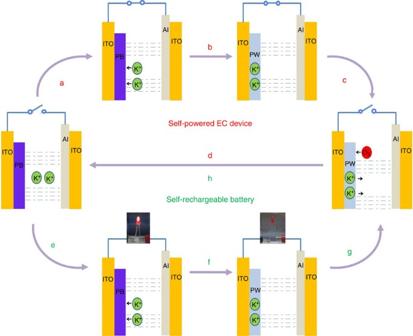Figure 7: Schematic illustrations of functioning mechanisms for the bi-functional device. (a–d): the bleaching and recovery processes of the device serving as a self-powered EC device, (e–h): the discharging and self-recharging processes of the device functioning as a self-rechargeable battery. 7e,f ) of the PB/Al cell might be expressed by the following half-cell reactions: Figure 7: Schematic illustrations of functioning mechanisms for the bi-functional device. (a–d): the bleaching and recovery processes of the device serving as a self-powered EC device, (e–h): the discharging and self-recharging processes of the device functioning as a self-rechargeable battery. Full size image The overall cell reaction can be expressed as: Reaction (3) is a typical half-cell reaction of a primary battery. Reaction (4) shows the reduction of PB to PW, which is similar to insertion-type reaction in a lithium battery. The as-prepared PB/Al cell combines the characteristics of primary battery and lithium battery. The output voltage of this PB/Al cell (1.26 V) is sufficient to drive the switching from PB to PW ( Fig. 7b ). For the recovery as a self-powered EC device ( Fig. 7c,d ) or charging as a self-rechargeable battery ( Fig. 7g,h ) of the PB/Al cell, oxygen plays a key role by oxidizing Fe(II) in PW to Fe(III) to form PB, in which the inserted K + ions are simultaneously extracted from PW. This interesting chemical property of PW, that is, spontaneously reverting to PB in the presence of oxygen [19] , [32] , has not previously attracted significant attention. Moreover, it is even generally regarded as a drawback in making a battery because it causes a reduction of the battery voltage [27] , and as a result, the battery needs to be isolated from air. However, here we make good use of this interesting property to prepare a self-rechargeable battery. The bleached device recovers its colour after oxidation by oxygen in air; the process ( Fig. 7g,h ) might be described by the following reaction: OH − ions generated by Reaction (6) will react with Al 3+ ions from Reaction (3) to form Al(OH) 3 precipitate, which has indeed been observed in our experiment. As a result, the pH value of the electrolyte remains stable, ensuring the reversibility of bleaching/colouration (as a self-powered EC device) and charging/discharging (as a self-rechargeable battery) of the as-prepared PB/Al cell. The consumption of Al is negligible because the PB film used in the cell is very thin with a tiny mass. Considering the critical role of oxygen, the recovery rate of the PB/Al cell may be further improved by increasing the open area of electrolyte to air or designing oxygen flow into the electrolyte. The PB/Al cell reported here is quite different from aluminium-air [36] or lithium-air [37] , [38] , [39] batteries in which Al or Li serves as the anode and O 2 serves directly as the cathode. Whereas in the PB/Al cell, PB serves the cathode during the discharging process and O 2 is only involved in the self-charging process. Lastly, it should be pointed out that when Al is eventually used up completely, the battery will not function any more. However, since Al is far in excess, in the reasonable lifetime of a normal rechargeable battery, the PB/Al battery demonstrated here is ‘self-rechargeable’ although a truly self-rechargeable battery cannot exist in reality from the first law of thermodynamics. A bi-functional PB/Al device has been demonstrated for self-powered EC window and self-rechargeable transparent battery. Without applying any external bias, PB can be bleached to PW by connecting the PB and Al electrodes. After bleaching, the blue colour of PB can be spontaneously recovered with PW oxidized by oxygen in air. In this regard, the designed PB/Al cell can be used as an energy-saving EC smart window which requires no external power source. The as-prepared PB/Al cell can also be used as a battery with a high output voltage. Most importantly, after discharging, such a battery can automatically self-recharge, that is, re-gaining the PB cathode voltage by reacting with oxygen in air. The discharging and charging of the self-rechargeable battery correspond to the bleaching and colouration of the self-powered EC device, respectively. Fast charging (4.6 s) of the battery can be realized by employing an external bias of 2 V. The as-prepared device exhibits promising applications in broad fields, for example, as a self-powered smart window to perform indoor light and heat management, and as a self-rechargeable transparent battery to power some delicate devices. Preparation of PB film ITO-coated glass with dimensions of 50 × 50 mm 2 was sequentially washed by deionized water, acetone, isopropanol and deionized water. After drying, three sides of the conductive surface of the ITO glass were covered by adhesive tape of size 50 × 5 mm 2 , keeping one side uncovered. PB film was prepared by electrochemical deposition on ITO glass (20 Ω/square), using the modified Neff method [21] . The electrolyte for PB electrochemical deposition is a mixed aqueous solution containing 10 mmol l −1 K 3 [Fe(CN)] 6 , 10 mmol l −1 FeCl 3 and 50 mmol l −1 KCl. The electrochemical deposition was carried out by a three-electrode electrochemical cell using a Potentiostat (VersaSTAT 3 F Potentiostat/Galvanostat, Princeton Applied Research), under a constant current density of −50 μA cm −2 for 300 s. The as-prepared PB film has an optimal contrast switch and a thickness of ~450 nm. ITO glass, Pt sheet and Ag/AgCl were used as the working electrode, counter electrode and reference electrode, respectively. Preparation of PB/Al device A slim Al sheet with dimensions of 60 × 5 mm 2 was attached onto one side of the conductive surface of another piece of ITO glass. A box-like EC device was fabricated by assembling the ITO glass deposited with PB film, ITO glass attached by Al sheet, common glass slides of size 50 × 7 mm 2 using epoxy. Thus, the spacing between two electrodes (PB film and Al sheet) is determined by the width of the common glass used in the device. The electrolyte (3 mol l −1 KCl aqueous solution) was dropped into the device. The mass loading of PB on ITO glass is about 65.5 μg cm −2 . Property characterization The transmittance spectra of the device before and after switching were measured by an ultraviolet–visible spectrophotometer (JESCO V670). Electrochemical measurements were carried out using a potentiostat (VersaSTAT 3 F Potentiostat/Galvanostat) and a CHI 660D electrochemical workstation. Electrochemical measurements were conducted in either a two-electrode configuration or a three-electrode configuration at room temperature using a 3 mol l −1 KCl aqueous solution as electrolyte. For the two-electrode configuration, PB film on ITO glass was used as the working electrode and Al foil serves as the counter electrode. For the three-electrode system, Al foil and SCE were used as the counter electrode and the reference electrode, respectively. The electrochemical measurements using the two-electrode configuration were performed in a voltage range of 0.8−2.1 V. Meanwhile, for the three-electrode system, the voltage range is −0.3–1.2 V. Electrochemical impedance spectroscopy measurements were carried out by applying an AC voltage with 1 mV amplitude in a frequency range of 0.1 Hz–100 kHz at open circuit potential in the three-electrode configuration. How to cite this article : Wang, J. et al. A bi-functional device for self-powered electrochromic window and self-rechargeable transparent battery applications. Nat. Commun. 5:4921 doi: 10.1038/ncomms5921 (2014).